Local adaptation limits lifetime reproductive success of dispersers in a wild salmon metapopulation Demographic and evolutionary dynamics in wild metapopulations are critically affected by the balance between dispersal and local adaptation. Where populations are demographically interconnected by migration, gene flow is often assumed to prevent local adaptation. However, reduced fitness of immigrants may limit gene flow between populations adapted to distinct habitat types, although direct quantification of the lifetime reproductive success of immigrants in the wild is lacking. Here, we show that dispersers between stream-spawning populations of sockeye salmon ( Oncorhynchus nerka ) had similar reproductive success to those that spawned in their natal stream, whereas dispersers from a different habitat (nearby lake beaches) produced half as many offspring. The stream- and beach-spawning ecotypes exhibited striking morphological differences despite their close spatial proximity, yet dispersal from the beach to the streams was more common than dispersal between streams, presenting empirical evidence that variation in immigrant reproductive success is important for the maintenance of intraspecific biodiversity. Local adaptation influences both ecological (distribution, productivity, resilience) and evolutionary (genetic diversity and divergence) properties of population complexes and species [1] . Theoretical work has found that gene flow and habitat-specific selection can interact in complex ways to influence local adaptation [2] , but empirical studies of wild interconnected populations have rarely been able to untangle the various mechanisms involved. For example, negative correlations between adaptive divergence and estimates of gene flow are commonly observed (‘isolation by adaptation’) [3] , but the causality of that relationship is not obvious as local adaptation may limit gene flow and vice versa [4] . The interaction between gene flow and local adaptation is particularly relevant in metapopulations occupying heterogeneous habitats [5] . A metapopulation is a group of spatially discrete, partially ephemeral populations that exchange dispersers [6] , and high dispersal rates can be favored when local population extinctions are common [7] . Thus, gene flow could be expected to prevent local adaptation in highly dynamic metapopulations. However, even in the presence of considerable dispersal, gene flow may be limited if dispersers have low reproductive success in already occupied habitats. Where local adaptation has arisen, dispersers between populations occupying distinct habitat types will be maladapted to their new habitat compared with philopatric (non-dispersing) individuals and dispersers between similar habitats, reducing gene flow and reinforcing local adaptation [8] , [9] . Empirical measurements of the relative reproductive success of dispersers between ecologically distinct habitats, however, have proven elusive. Reciprocal translocation experiments have often (but not always) shown that survival and fecundity are higher in philopatric individuals than immigrants [10] , [11] , [12] , [13] . However, most of these studies did not measure reproductive success (and thus fitness), and typically used randomly selected individuals as ‘immigrants’ whereas natural dispersers may differ phenotypically and genetically from their philopatric conspecifics [14] . Furthermore, information on phenotypic and habitat differences between populations is generally missing, complicating the interpretation of results. Alternatively, indirect estimates of gene flow can be relatively easily obtained from genetic differentiation, but only under stringent assumptions on population structure and evolutionary equilibria that are unlikely to be fulfilled in most wild populations [15] . Direct, simultaneous measurement of dispersal rates and the reproductive success of dispersing individuals in the wild can be achieved by pedigree reconstruction. However, few studies employing this labour-intensive technique have attempted to identify the natal origins of immigrants; most have grouped all individuals not native to the focal population into a single category, ignoring the diversity of source populations that could contribute to the immigrant group [16] , [17] . Without comparisons between immigrants from different habitat types, it is impossible to separate the fitness effects of dispersal itself (for example, precedence and familiarity) from the effects of local adaptation. In an exceptional study, great reed warbler immigrants from distant populations had lower reproductive success than immigrants from nearby populations [18] , suggesting that not all dispersers experience the same fitness consequences. Nevertheless, geographical distance is not a good proxy for adaptive divergence between subpopulations, so the relationship between local adaptation and reproductive success of dispersers remains unresolved. Pacific salmon frequently show local adaptation over small spatial scales [11] despite dispersal rates of 2–10% [19] . Well-characterized examples of this adaptive diversity are tributary stream-spawning and lake beach-spawning sockeye salmon ( Oncorhynchus nerka ) ecotypes [20] , [21] . Differences between these ecotypes in body size and shape [22] , egg size [23] and migration timing [24] are likely maintained by divergent natural and sexual selection regimes [22] . Dispersal between stream and beach-spawning habitats is relatively frequent, but dispersers are morphologically more similar to their recipient populations than expected under random dispersal, suggesting that dispersers may be somewhat pre-adapted to their chosen spawning habitat [25] . Importantly, because of anadromy and semelparity of Pacific salmon, philopatric individuals have no advantage over immigrants in terms of familiarity and precedence, an issue that has complicated interpretation in other studies. Here, we estimated the effect of local adaptation on gene flow by quantifying the relative fitness (that is, reproductive success) of philopatric and immigrant sockeye salmon in two stream-spawning populations in southwest Alaska (A and C Creeks; Fig. 1 ). Using genetic population assignment and pedigree reconstruction over two brood years, we compared the lifetime reproductive success of all philopatric fish, dispersers between creeks and dispersers from adjacent lake beaches. Rather than a general fitness cost of dispersal [16] , [17] , or of geographic distance between natal and spawning populations [18] , we found that local adaptation to specific habitat types limited the reproductive success of dispersers between ecologically distinct populations. The consequent restriction of gene flow between habitat types helps to explain the genetic, morphological and behavioural diversity observed over very small spatial scales in this system [22] , [24] , [25] . 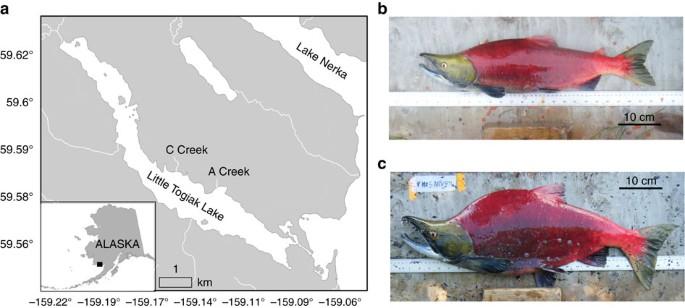Figure 1: Study sites and populations. (a) Map of study sites. Beach-spawning sites are located within 100 m of the mouth of each creek. Square in inset map indicates location within Alaska. (b) Representative male of the stream-spawning ecotype. (c) Representative male of the beach-spawning ecotype. Photographs courtesy of Wesley A. Larson. Figure 1: Study sites and populations. ( a ) Map of study sites. Beach-spawning sites are located within 100 m of the mouth of each creek. Square in inset map indicates location within Alaska. ( b ) Representative male of the stream-spawning ecotype. ( c ) Representative male of the beach-spawning ecotype. Photographs courtesy of Wesley A. Larson. Full size image Population sizes and differentiation We tagged and sampled a total of 4,473 individuals in A Creek and C Creek in 2004, 2005, 2008, 2009 and 2010, and 166 individuals that settled on the beach habitat in 2004 and 2005. The overall sex ratio of all individuals sampled in this study was 66% female, ranging from 58–71% over populations and years. Genetic differentiation (pairwise F ST ) between populations ranged from 0.017–0.039 ( Table 1 ). Table 1 Genetic differentiation of sampled populations. Full size table Genotyping and error checking Of the 4,639 individuals sampled, 4,377 were fin-clipped and 4,350 were successfully genotyped at eight or more loci. Twenty-seven individuals genotyped at fewer than 8 of 11 loci were removed from the data set because parentage assignments were not reliable in this group. Departures from Hardy–Weinberg equilibrium were found in 100 of the 132 tests, probably because of small population sizes. There was evidence for null alleles at three loci (One100a, One106 and One115a; as found by Hauser et al. [26] ). Linkage disequilibrium was statistically significant for all pairs of loci within each stream subpopulation, but only 3 of 55 locus pairs were significantly linked in the beach population. Estimated effective population sizes ( N e ) were lower for the stream subpopulations than for the beach subpopulation. The ratios of the estimated N e values to the census sizes (0.13–0.44) are similar to those reported for other salmonid populations [27] , suggesting that the observed linkage is caused by small N e rather than physical linkage between loci. Individual genotype and tagging data have been deposited in Dryad ( www.datadryad.org ). Identification of dispersers Individuals genetically assigned to all three potential source populations were sampled in both streams in 2004 and 2005 ( Supplementary Table 1 ), and 83% of assignments were given confidence scores of at least 95%. 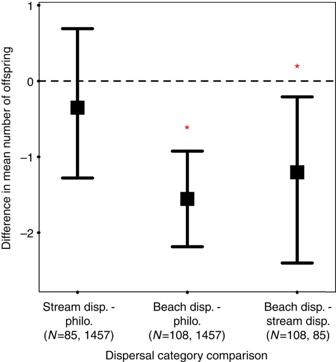Figure 2: Differences between dispersal categories in mean reproductive success. Values represent the model-predicted effect of dispersal category differences on number of offspring after accounting for differences in reproductive success between spawning streams, sexes and spawning years. Error bars indicate 95% confidence intervals (CIs). * indicates a difference that is statistically significant after bootstrapping (95% CI does not include zero). Philo., philopatric individuals; stream disp., between-stream dispersers; beach disp., beach-to-stream dispersers. Immigrants (fish assigned to a population other than the one in which they were captured) made up 3–28% of populations in the streams depending on sex, spawning year and spawning stream (12% overall; Table 2 ). C Creek had more immigrants from the other stream as well as from the beach than A Creek, but there was no clear sex bias in dispersing individuals. The number of individuals immigrating from the beach-spawning populations ( N =108) was greater than the number of dispersers between stream-spawning populations ( N =85). Simulations suggested that 88–95% of our population assignments were correct, depending on population of origin ( Supplementary Table 2 ). Table 2 Population assignments by sex – 2004–2005. Full size table Between-stream dispersers were morphologically similar to philopatric individuals, but immigrants from the beach-spawning population were longer and deeper-bodied than creek fish ( Supplementary Figs 1 and 2 ). Beach-to-stream dispersers also had shorter in-creek residency periods than both philopatric fish and between-stream dispersers ( Supplementary Fig. 3 ), but beach-to-stream dispersers were less likely to be killed by bears and more likely to have an unknown fate ( Supplementary Fig. 4 ). Pedigree reconstruction Pedigree reconstruction identified 552 unique, confidently ( P >95%) assigned parent pairs (sire and dam) and 127 unique, confidently assigned single parents in 2004 and 2005. Only 17 parent-offspring assignments were discarded because of<95% confidence. Both parents were sampled in the same year in 96% of inferred triads (offspring and both parents) and in the same stream in 98% of triads. Of 711 F1 individuals sampled in 2008, 461 (65%) were assigned to a parent pair and 124 (17%) were assigned to a single parent. Of 1,167 F1 individuals sampled in 2009, 1,031 (88%) were assigned to a parent pair and 89 (8%) were assigned to a single parent. Of 725 F1 individuals sampled in 2010, 179 (25%) were assigned to a parent pair and 58 (8%) were assigned to a single parent, likely because the 4-year-old cohort (whose parents returning in 2006 were not genotyped) dominated in this year. Reproductive success Reproductive success was extremely variable among individuals, with the number of inferred offspring ranging from 0 to 36 (mean 3.4) for males and 0 to 24 (mean 1.6) for females ( Supplementary Table 1 ). No offspring were assigned to 49% of males and 68% of females. The reproductive success of dispersers between the two stream-adapted populations did not differ significantly from that of philopatric individuals, but immigrants from the beach population had significantly lower mean reproductive success than both philopatric fish and immigrants from the other stream ( Fig. 2 ). This difference was consistent over most combinations of sexes, spawning streams and spawning years when sample size was sufficient ( Fig. 3 ). On average, beach-to-stream dispersers produced about one fewer offspring than between-stream dispersers, a reduction in fitness equivalent to almost half (46%) of the average reproductive success. Detailed analysis of the zero-inflated regression results suggested that immigrants from the beach were more likely to be completely unsuccessful (that is, produce no offspring) and produced fewer offspring even when successful ( Supplementary Fig. 5 ). Figure 2: Differences between dispersal categories in mean reproductive success. Values represent the model-predicted effect of dispersal category differences on number of offspring after accounting for differences in reproductive success between spawning streams, sexes and spawning years. Error bars indicate 95% confidence intervals (CIs). * indicates a difference that is statistically significant after bootstrapping (95% CI does not include zero). Philo., philopatric individuals; stream disp., between-stream dispersers; beach disp., beach-to-stream dispersers. 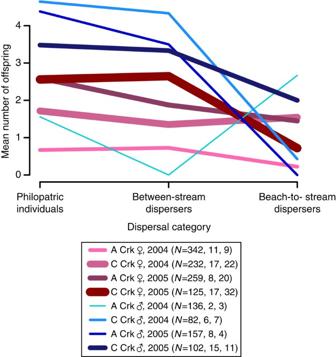Figure 3: Mean reproductive success by population. Thickness of lines is weighted by total sample size of creek and beach dispersers. A Crk, A Creek; C Crk, C Creek. Full size image Figure 3: Mean reproductive success by population. Thickness of lines is weighted by total sample size of creek and beach dispersers. A Crk, A Creek; C Crk, C Creek. Full size image Almost all reproductively successful dispersers mated with a philopatric individual rather than another disperser. Of 136 female and 56 male dispersers identified, 30 females and 18 males had at least one offspring, collectively participating in 91 inferred mate pairs. Of these successful dispersers, the ratio of beach-to-stream to between-stream dispersers was nearly equal (21:27). Only one mating event between dispersers was inferred, indicating that the proportion of successful disperser mating events that involved a philopatric mate was 0.99. A Fisher’s exact test provided no evidence for departure from random mating with respect to dispersal status ( P =0.92). Direct comparison of the lifetime reproductive success of dispersers within and between habitat types enabled us to assess the effect of local adaptation on gene flow in a metapopulation of sockeye salmon. Specifically, the reproductive success of immigrants from the beach population was just half that of philopatric creek-spawning fish and between-creek dispersers. Nevertheless, dispersal from beach to creek was at least as common as that between creeks. Although dispersers from the beach-adapted population to the creeks were somewhat deeper-bodied than other creek fish, they were less likely to be killed by bears and appeared to leave the creek voluntarily. The mechanism of reduction in reproductive success of beach dispersers therefore appeared to be more complex than direct bear predation. Morphological adaptation to the ecologically distinct habitat types may have been responsible for the observed differences in reproductive success between disperser categories. The two study streams are extremely shallow (~10 cm depth) and salmon have been found to be under intense, size-selective predation pressure from bears in similar habitats, benefitting shallower and smaller fish [28] . In lake beach habitats, however, fecundity, direct competition for mates and nest sites and relaxed predation pressure select for larger, deeper fish [22] . Although dispersers between the two habitats are not random representatives of their populations and tend to resemble the recipient populations [25] (for example, dispersers from the beach population were shallower than philopatric beach spawners), beach immigrants were nevertheless generally longer and deeper-bodied than stream-adapted fish. Physical maladaptation to the stream environment could limit the reproductive success of beach-adapted immigrants by reducing adult lifespan during the spawning period through selective bear predation or stranding in shallow water [29] . Moreover, reduced physical access to shallower areas of the stream could limit access to mates and spawning sites, reducing reproductive opportunities. The reproductive success of dispersers between habitat types may also have been limited by divergent selection on behavioural traits. The relatively large proportion of beach-to-stream dispersers that disappeared without a recorded death fate suggests that voluntary departure rather than bear predation was the mechanism limiting their in-stream residency period. These fish may have been searching for their natal habitat or ‘prospecting’ a novel habitat for potential spawning sites, a behaviour that has been observed in other sockeye salmon populations [30] . Nevertheless, these individuals should be considered dispersers because they were sexually mature, competed for space and possibly for mates, and may have reproduced in the streams. Indeed, beach-to-stream dispersers produced fewer offspring than between-creek dispersers and philopatric fish even after accounting for the individuals that did not reproduce at all. Furthermore, even philopatric fish show a wide variety of movement strategies, and recent PIT tagging work in A and C Creeks suggests that many fish may move between stream and lake on a daily basis [31] . There is therefore wide individual variation in movement strategies, which may have a genetic basis or represent plastic responses to individual predation vulnerability. Bears may therefore indirectly affect reproductive success by eliciting predator avoidance behaviour and thereby limiting reproductive opportunity. Thus, adaptive behavioural differences between ecotypes may strongly influence the conversion of dispersal into gene flow. In addition to limited mating success of the spawning adults, viability selection against the offspring of immigrants from the beach-spawning population could have contributed to the reduction in returning adult offspring of dispersers between habitat types. Nearly all reproductively successful immigrants mated with a philopatric individual, producing potentially maladapted hybrid offspring. However, juveniles from both stream- and beach-spawning populations congregate in the lake immediately after emergence from the gravel [32] , so opportunities for habitat-specific selection after mating are limited to the incubation and emergence life stages. Our study provides clear empirical evidence of gene flow limited by ecotype-specific disperser reproduction rather than by barriers to dispersal between habitat types. Beach-to-stream dispersers were more common than between-stream dispersers, suggesting that dispersal between habitat types is not restricted by intrinsic or extrinsic barriers. The high cost of local adaptation to dispersers, roughly half of an individual’s expected reproductive output, may therefore be crucial to the maintenance of the morphologically and genetically recognizable stream- and beach-spawning ecotypes. Although low fitness of dispersers might be expected to drive the evolution of intrinsic barriers to dispersal in some systems [8] , additional factors may select against such barriers. For example, in dynamic metapopulations, rare subpopulation recolonization events may substantially bolster the long-term fitness of dispersal alleles even if dispersers have limited reproductive success in occupied subpopulations [7] . Moreover, flexible behaviour patterns in systems that allow for reversal of dispersal decisions could minimize the fitness cost of dispersal in unfavourable conditions [33] . Thus, in many metapopulations, reduced immigrant reproductive success may be more important than barriers to dispersal for the maintenance of intraspecific biodiversity. A metapopulation in which gene flow is reduced by local adaptation rather than dispersal limitation may respond more quickly to changes in selective regimes due to climate cycles or anthropogenic impacts because genotypes from pre-adapted, productive populations will rapidly invade other populations [34] . Furthermore, mechanisms that reduce but do not eliminate gene flow between divergent populations can maintain local adaptation and functional diversity while also allowing rapid spread of novel advantageous alleles [2] . Sample collection Exhaustive sampling of A and C Creek adult spawning populations was conducted every year from 2004 through 2010. Fish were tagged with coloured Petersen disc tags with individual two-letter codes. We walked the full length of both streams every day during the spawning season (late July through late August), tagging any newly observed (that is, untagged) fish and noting the location of each previously tagged fish. To expedite tagging during times of peak abundance, fish in the lake at the mouth of each stream were captured by beach seine and tagged before they entered the streams. A fin clip was taken from each fish upon tagging for genetic analysis. Sex, body length (mid-eye to hypural plate), and body depth (anterior insertion of the dorsal fin to the belly) were also measured and recorded for each newly tagged individual [22] . When a dead fish was found in or near either stream, the tag ID was recorded and the cause of death was determined by visual inspection (mostly either bear kill or senescence). If a dead fish was found untagged, a fin clip was taken and length and depth were measured if the carcass was intact. Fish present on the beach-spawning habitats adjacent to A and C Creeks were captured with a beach seine on a weekly basis throughout the spawning season. Laboratory methods All adults observed in either A or C Creek in 2004, 2005, 2008, 2009 and 2010 were genotyped at 11 tetranucleotide repeat microsatellite loci (mean expected heterozygosity in all samples=0.87±0.04 s.d., 266 independent alleles; Supplementary Table 1 ). All individuals sampled after they had settled on redds (nests) in the beach habitats in 2004 and 2005 were also genotyped to provide a genetic baseline for identification of dispersers in the F0 generation. DNA was extracted from the samples using Qiagen DNeasy extraction columns following the manufacturer's instructions. Microsatellite loci were amplified in three multiplex panels using Qiagen multiplex PCR kits, with varying primer concentrations and annealing temperatures ( Supplementary Tables 3 and 4 ). Forward primers were fluorescently labelled and amplified fragment sizes were measured with a MegaBACE 1000 DNA Analysis System (GE Healthcare Life Sciences). To quantify genotyping error rates, 146–203 individuals were re-amplified and re-genotyped at each locus. Pedigree reconstruction Parent-offspring relationships between the F0 generation (stream spawners in years 2004 and 2005) and their F1 offspring (stream spawners in years 2008–2010) were reconstructed using the parentage analysis software package Colony v2.0 (ref. 35) [35] . All genotyped F0 individuals were considered to be either potential dams or sires (according to their observed sex) for all genotyped F1 offspring, and F0 individuals of unknown sex were included as both potential dams and potential sires. Data from both stream populations and all years were incorporated into a single pedigree reconstruction to account for dispersal between streams in the offspring generation, as well as the variation in age-at-return of those offspring. Individuals that spawned on the beach were not included in the parentage reconstruction because dispersal between beach-spawning habitats in the lake is too high to allow comprehensive sampling of potential parents. Only parent-offspring relationships with a confidence score greater than 95% were included in subsequent analyses. From this confidently assigned subset of the pedigree, the total number of stream-spawning offspring assigned to each F0 individual was tabulated. Colony accounts for the fact that not all parents may be sampled, and we conservatively set the estimated probability of a stream-spawning parent being sampled at 0.7, the proportion of adults sampled in 2008 assigned to parents that were sampled in 2004 in the A Creek population by Hauser et al. [26] A sensitivity analysis of the proportion of sampled parents indicated that this parameter had negligible effects on the parentage assignments. Identification of dispersers The spawning location of each individual in the parental generation was inferred from field observations. Fish that entered a single stream were classified as A or C Creek spawners, depending on the stream where they were observed. If a fish entered both streams, the stream in which it was seen more often was considered to be its chosen spawning habitat. The accuracy of these spawning location classifications was assessed by comparing the spawning locations of mates inferred by parentage analysis. Fish that never entered either stream but were observed on redds on the beach were classified as beach spawners. The most likely natal population for each individual in the parental generation was estimated using a Bayesian genetic assignment method [36] implemented in the software GeneClass2 (ref. 37) [37] . F0 genotypes were grouped into A Creek, C Creek and beach populations based on the observationally inferred spawning location of each individual. We considered the two sampled beach-spawning sites as one population because beach-spawning aggregations throughout the entire lake exhibit very low genetic and morphological differentiation [25] . A leave-one-out procedure was utilized to assign each individual to its most likely natal population [37] , with the two stream populations and the beach population considered as the only potential natal populations. The number of immigrants from un-sampled populations in our sample was likely small because A and C Creeks are the only streams consistently used by salmon in Little Togiak Lake, and because the beach population is effectively panmictic. Dispersal status for each stream-spawning individual was determined by comparing its genetic population assignment with its inferred spawning location. Fish were classified as philopatric if they spawned in the stream of their natal population assignment, between-stream dispersers if they spawned in the stream that was not assigned as their natal population, and beach-to-stream dispersers if they spawned in either stream but were genetically assigned to the beach population. The accuracy of the assignment method was assessed by simulation: 10 pools of simulated genotypes of the same size as the original data set were produced and source populations were assigned to each individual using the leave-one-out Bayesian assignment method. Simulated genotypes were produced by combining multilocus haploid ‘gametes’ from random individuals within each population, thereby preserving any linkage disequilibrium present in the data [38] . The assignment algorithm in GeneClass2 produces a probability of each multilocus genotype belonging to each population, which was used as a confidence score for each assignment. The accuracy of the assignment method for simulated individuals from each population was quantified by calculating the proportion of individuals assigned to each of the three populations under two approaches: (1) accepting the most likely population of origin for each individual regardless of statistical confidence and (2) only accepting the most likely population of origin when it was assigned with 95% confidence interval or greater. Because of the likelihood that philopatric fish would greatly outnumber dispersers, we were concerned that even low misassignment rates of philopatric individuals could produce a large ratio of spurious dispersers to true dispersers. We therefore conducted a second verification of the dispersal category assignment method by comparing the results of population assignments in an offspring cohort with the results of our parentage analysis. Parentage reconstruction is often a much more accurate method to identify dispersers (in the offspring generation) between genetically similar populations than population assignment tests [39] , so it offers an excellent empirical assessment of the validity of our dispersal assignments [40] . We compared parentage with dispersal assignments in the 2009 cohort because both 4- and 5-year-old fish should have sampled parents (2004 and 2005), and so almost all fish should have parents assigned if they spawned in the streams. We therefore evaluated the accuracy and power of the dispersal categories inferred from the population assignment method by calculating, for each assigned dispersal category, the number of individuals with two parents from the same stream (true philopatric individuals), two parents from the other stream (true stream-to-stream dispersers) or zero parents assigned (either true immigrants from the beach population or offspring with neither stream-spawning parent sampled). Parents were expected to be from the same creek for putative philopatric individuals and from the other stream for putative stream dispersers. No parents were expected to be assigned for putative beach dispersers. Offspring were included only if they were sampled in A or C Creek and had neither or both parents assigned. Our results indicated that using the 95% confidence assignment cutoff produced dispersal category assignments with a higher proportion of individuals with parents that spawned in the expected locations ( Supplementary Fig. 6 ). However, this increased accuracy came at the cost of sample size–many true dispersers were eliminated by the cutoff, particularly those from the beach population. Because we did not expect a bias from misassignments, but only a decrease in power to differentiate reproductive success between dispersal categories, we ran further analyses using the full data set. Nevertheless, using the assignment cutoff does not substantially affect the results ( Supplementary Fig. 7 ). Comparison of dispersal groups in morphological and behavioural traits The three dispersal groups were compared in the following traits: sex ratio, body length, body shape (body depth/body length ratio [41] ), residency period on the spawning grounds (total number of days observed in the stream) and death fate (bear-killed, senescent or unknown). The data set was divided by sex and stream to create four groups, within each of which trait distributions were compared between dispersal categories. Significant differences between dispersal categories in mean trait values were evaluated with Fisher’s exact tests for categorical variables and generalized linear models (GLMs) for continuous variables. In the case of the GLMs, the morphological or behavioural trait of interest was the response variable and dispersal category was the predictor variable. The best distribution for each continuous trait was chosen by evaluating the Akaike information criterion (AIC) for models assuming normal, Poisson and gamma distributions and a simple intercept as the only predictor. The gamma distribution produced the lowest AIC for all traits. Comparison of reproductive success between dispersers and philopatric individuals The relationship between individual dispersal status and reproductive success was characterized with zero-inflated negative binomial (ZINB) regression models to accommodate the distribution of the response variable, reproductive success [42] . Validation of this model choice using AIC values indicated that the ZINB model provided a better fit to the data than a standard GLM with a normal or Poisson distribution. ZINB regression models were implemented with the ‘pscl’ package v1.04.1 (ref. 42) [42] implemented in the R statistical environment v2.13.2 (ref. 43) [42] . We used the ZINB model to quantify the difference between dispersal groups in reproductive success: the response variable was the total number of offspring per F0 individual and the predictor variable of interest was dispersal category (philopatric, between-stream disperser or beach-to-stream disperser). We also included sex, spawning stream and spawning year as additional fixed factors. All pairwise interactions between these four categorial variables were evaluated for inclusion in the model using a stepwise model selection procedure [44] . The resulting model was used to calculate the difference in mean number of offspring between dispersal categories after accounting for the effects of sex, spawning population and year. Statistical confidence in the differences in reproductive success between dispersal categories was assessed by bootstrapping individuals in each dispersal category per sex and stream, re-parameterizing the regression model and recalculating differences between groups 1,000 times. Differences in reproductive success were considered statistically significant if the range between the 2.5 and 97.5% quantiles of the estimates did not include zero [45] . This model was run both with and without a 95% assignment confidence cutoff, but using the cutoff did not substantially affect the parameter estimates, although confidence intervals were larger due to the smaller sample sizes ( Supplementary Fig. 7 ). Mate choice with regard to dispersal status We determined whether reproductively successful dispersers mated with other dispersers or with philopatric individuals. We therefore calculated the proportion of successful dispersers that mated with another disperser. To test whether the observed pattern was significantly different from expectations under random mating, we performed a Fisher’s exact test on a table of the number of inferred matings between males and females from each dispersal category. How to cite this article: Peterson, D. A. et al. Local adaptation limits lifetime reproductive success of dispersers in a wild salmon metapopulation. Nat. Commun. 5:3696 doi: 10.1038/ncomms4696 (2014).